Chiral phosphoric acid catalyzed aminative dearomatization ofα-naphthols/Michael addition sequence Asymmetric dearomatization reactions have recently emerged as a powerful tool for the rapid build-up of the molecular complexity. Chiral three-dimensional polycyclic molecules bearing contiguous stereogenic centers can be synthesized from readily available planar aromatic feedstocks. Here we report that an intermolecular asymmetric dearomatization reaction of α -naphthols bearing a tethered nucleophile at the C4 position of the naphthol ring is achieved by a chiral phosphoric acid. The reaction proceeds via a highly chemo- and regioselective aminative dearomatization/Michael addition sequence, affording a wide array of functionalized cyclic ketones in good yields (up to 93%) with excellent enantioselectivity (up to >99% ee). The catalyst loading can be reduced to 0.1 mol%. Preliminary mechanistic investigations identify that the enantioselectivity is established in the dearomatization step, while the Michael addition is the rate-limiting step. A working model accounting for the origin of the stereochemistry is proposed based on DFT calculations. The demands for effective assembly of diverse molecular scaffolds are continuously growing along with the development of organic chemistry. Among various kinds of strategies that aim to rapidly increase molecular complexity, catalytic asymmetric dearomatization (CADA) reactions [1] , [2] , [3] , [4] , [5] , [6] , [7] , [8] , [9] , [10] , [11] , [12] have recently received considerable attention of the synthetic community. They are capable of significantly enriching the chemical space by converting readily available planar aromatic compounds to diverse three-dimensional molecules bearing spiro or fused polycyclic skeletons with multiple stereogenic centers including quaternary ones. Naphthols serve as important aromatic feedstocks in organic chemistry. However, the asymmetric dearomatization reactions of naphthols are relatively less explored compared with those of other electron-rich arenes like indoles [13] , [14] , [15] , [16] , [17] , [18] . With the oxidation system consisting of a chiral hypervalent iodine reagent and m -CPBA as the terminal oxidant [19] , [20] , [21] , [22] , [23] , [24] , [25] , [26] , [27] , [28] , [29] , or transition-metal catalysts that are capable of promoting single electron oxidation [30] , [31] , α - or β -naphthols could react with intra- or intermolecular nucleophiles to yield chiral functionalized cyclic ketones. Notably, the asymmetric dearomatization reactions under non-oxidative conditions are rather limited within β -naphthols [32] , [33] , [34] , [35] , [36] , [37] , [38] , [39] , [40] , [41] , [42] , [43] , [44] , [45] , [46] , [47] , [48] , [49] , [50] , [51] , [52] , and the corresponding reactions of α -naphthols are relatively rare. In 2015, Luan and coworkers reported an elegant Pd-catalyzed dynamic kinetic asymmetric transformation of 4-(2-bromoaryl)- α -naphthols with alkynes for the synthesis of chiral spirocyclic enones [53] . Sporadic examples of non-oxidative asymmetric dearomatization of α -naphthols via organocatalytic chlorination [37] , annulation [54] , Ir-catalyzed allylic alkylation [38] , or Pd-catalyzed cross coupling [55] , [56] , [57] were disclosed. However, the dearomatization reactions in these examples generally relied on the pre-installation of an intramolecular electrophile (Fig. 1a ). Notably, during the preparation of this manuscript, Shao and coworkers reported an intermolecular asymmetric allylic dearomatization reaction of α -naphthols at the C2 position by a chiral phosphoric acid [58] . However, highly efficient asymmetric dearomatization reactions of α -naphthols with intermolecular electrophiles still remain underdeveloped. Fig. 1 Catalytic Asymmetric Dearomatization of α -Naphthols at the C4 Position. a Intramolecular dearomatization. b Intermolecular sequential dearomatization/Michael addition. Ar: aromatic ring, El: electrophile, Nu: nucleophile, R: substituent Full size image In 2017, we reported a Pd-catalyzed arylative dearomatization/ aza -Michael addition sequence between aryl bromide and α -naphthols bearing a tethered nucleophile at the C4 position of the naphthol ring [59] . The exclusive chemo-, and regioselectivity favoring the C4 position among the multiple potential nucleophilic sites encouraged us to further probe the possibility of developing a highly enantioselective dearomatization of α -naphthols/Michael addition sequence. However, all attempts to realize such an asymmetric reaction under Pd catalysis have been failed in our hands. In this regard, we speculated that azodicarboxylates [60] , [61] , [62] , [63] , [64] , [65] , [66] might be employed as suitable electrophilic amination reagents which are compatible with the dearomatization of electron-rich arenes in the presence of a chiral phosphoric acid (CPA) [67] , [68] , [69] , [70] . Here, we accomplished the efficient synthesis of a wide array of functionalized cyclic ketones bearing two consecutive stereogenic centers in excellent diastereo- and enantioselectivity (Fig. 1b ). The products are readily involved in further transformations towards various enantioenriched polycyclic molecules. 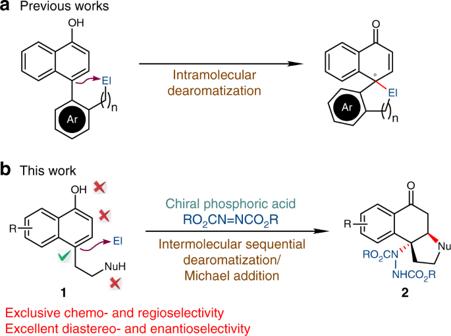Fig. 1 Catalytic Asymmetric Dearomatization ofα-Naphthols at the C4 Position.aIntramolecular dearomatization.bIntermolecular sequential dearomatization/Michael addition. Ar: aromatic ring, El: electrophile, Nu: nucleophile, R: substituent Reaction development Our studies commenced with the attempt of the reaction of α -naphthol 1a with 1.5 equivalents of diethyl azodicarboxylate (DEAD) (Table 1 ). In the presence of 10 mol% of chiral phosphoric acid C1 , the target reaction proceeded smoothly in 1,2-dichloroethane (DCE) at 50 °C for 24 h, affording the dearomatized product 2a in 85% yield with 75% ee as a single trans diastereoisomer (Table 1 , entry 1). The structure and absolute configuration of 2a (3 R ,4 R ) were established unambiguously by X-ray crystallographic analysis of an enantiopure sample. Interestingly, the Friedel–Crafts reaction at the C2 position was not observed. Systematic evaluation of a series of CPAs ( C2 – C7 ) was conducted (Table 1 , entries 2–7). The results revealed that the catalysts have great influence on the reaction outcome. Notably, TRIP-CPA C2 gave the optimal results (90% yield and 99% ee, Table 1 , entry 2). Utilizing SiPh 3 -derived catalyst C4 also led to comparable results with those of C2 (90% yield and 98% ee, Table 1 , entry 4). On the other hand, 2a was obtained in the nearly racemic form (2% ee) when 4-NO 2 C 6 H 4 derived C6 was employed (Table 1 , entry 6). Although excellent enantioselectivity has been obtained, other reaction parameters were further investigated. Typical solvents including EtOAc, THF or toluene also well facilitated the reaction (Table 1 , entries 8-10). When the temperature was lowered to 40 °C, prolonged time (36 h) was necessary to provide 2a in 88% yield (Table 1 , entry 11). Similar results (85% yield and 99% ee) could be achieved in shorter time when elevating the reaction temperature to 60 °C (Table 1 , entry 12). However, slightly decreased yield (77%) was observed when 1.1 equivalents of DEAD was used (Table 1 , entry 13). The reactions proceeded well with reduced loading of C2 (≤1 mol %, Table 1 , entries 14-17). The remarkably high catalytic efficiency was exemplified by the fact that 2a was afforded in 52% yield with 97% ee in the presence of 0.1 mol% of C2 at 80 °C (Table 1 , entry 17). 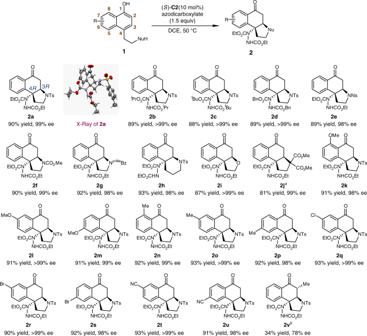Fig. 2 Substrate Scope ofα-Naphthols. Reaction conditions:1(0.1 mmol), azodicarboxylate (0.15 mmol) and (S)-C2(10 mol%) in DCE (2 mL) at 50 °C.aAfter work up,tBuOK (2 equiv in THF) was added at rt.bAt 0.2 mmol scale. Bz, benzoyl However, only complex mixture was obtained in the absence of a CPA catalyst (Table 1 , entry 18). Table 1 Optimization of the reaction conditions a Full size table Scope and limitation With the optimal conditions in hands (Table 1 , entry 2), we next explored the substrate scope (Fig. 2 ). The desired reactions of 1a with other azodicarboxylates all proceeded smoothly, leading to 2b – 2d in high yields (88–89%). The N -protecting group of α -naphthol substrates could be switched to Ns, CO 2 Me or p -MeC 6 H 4 CO 2 . The corresponding products ( 2e – 2g ) could be obtained in 89–92% yields. The prolonged tether at the C4 position of the naphthol ring was well accommodated, affording the piperidine-fused product 2 h in 93% yield. Besides nitrogen nucleophiles, the hydroxyl group could also work as the nucleophile. The tetrahydrofuran-fused product 2i was accomplished smoothly in 87% yield. Notably, when a malonate diester nucleophile was employed, only the dearomatization process occurred under the standard conditions. The target product 2j could be obtained (81% yield) after a subsequent Michael addition promoted by t BuOK. Fig. 2 Substrate Scope of α -Naphthols. Reaction conditions: 1 (0.1 mmol), azodicarboxylate (0.15 mmol) and ( S )- C2 (10 mol%) in DCE (2 mL) at 50 °C. a After work up, t BuOK (2 equiv in THF) was added at rt. b At 0.2 mmol scale. Bz, benzoyl Full size image On the other hand, various substituted α -naphthols underwent the desired dearomatization reactions. Electron-donating groups such as MeO and Me could be tolerated at the C6 to C8 positions ( 2k–2p , 91–93% yields). The C6 and C7 positions could accommodate halogen atoms including Cl and Br ( 2q–2s , 90–93% yields). Besides, when a CN group was installed at the C6 or C7 position, the dearomatization reaction delivered the desired products in high yields ( 2t , 93% yield; 2 u , 91% yield). Gratifyingly, exceedingly high enantioselectivity was observed in all the above cases ( 2a–2u , 98 to >99% ee). However, when the substrate bearing a methyl group at the C2 position was subjected to the standard conditions, the reaction outcomes decreased apparently in terms of yield and enantioselectivity ( 2v , 34% yield and 78% ee). It should be noted that only complex mixtures were obtained when substrates bearing a substituent at the C5 position were utilized. The dearomatization reaction of phenols is much more challenging compared with that of naphthols. In addition, by-products of Friedel–Crafts reactions are difficult to be avoided. To further expand the substrate scope of this aminative dearomatization/Michael addition sequence, several phenol analogs were tested (Fig. 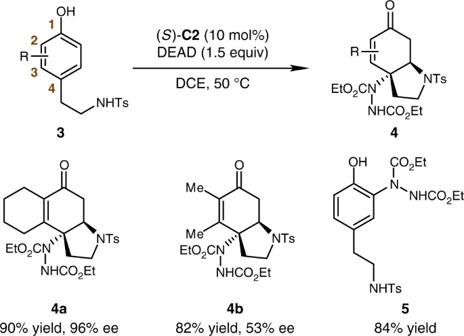Fig. 3 Substrate Scope of Phenols. Reaction conditions:3(0.1 mmol), DEAD (0.15 mmol) and (S)-C2(10 mol%) in DCE (2 mL) at 50 °C. Me, methyl 3 ). Encouragingly, α -tetrahydronaphthol-derived substrate 3a participated the title reaction smoothly, delivering the desired product 4a in 90% yield with 96% ee, without the observation of Friedel–Crafts by-product. The reaction of sterically less demanding phenol substrate (2,3-Me 2 ) also proceeded well. The corresponding product 4b was obtained in good yield (82%) but with rather decreased enantioselectivity (53% ee). Notably, a mixture of Friedel–Crafts-type byproducts became dominating for the substrates bearing one substituent (Me, MeO, or Br) at the C2 or C3 position. Compound 5 was isolated in 84% yield for the phenol substrate bearing no substituent at the C2 or C3 position. Fig. 3 Substrate Scope of Phenols. Reaction conditions: 3 (0.1 mmol), DEAD (0.15 mmol) and ( S )- C2 (10 mol%) in DCE (2 mL) at 50 °C. 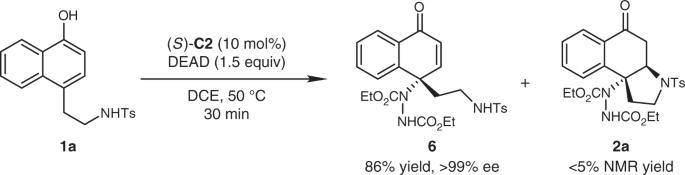Fig. 4 Isolation of the Intermediate. Reaction conditions:1a(0.1 mmol), DEAD (0.15 mmol) and (S)-C2(10 mol%) in DCE (2 mL) at 50 °C for 30 min Me, methyl Full size image Mechanistic studies To shed light on the reaction mechanism, we first attempted to isolate the intermediate of this sequential reaction (Fig. 4 ). When the reaction of 1a was quenched within 30 min, only trace amount of 2a was observed (<5% NMR yield), while conjugated enone 6 was isolated in 86% yield with >99% ee. Compound 6 was found stable enough to be stored at −20 °C for weeks without apparent transformation into 2a or decomposition. Taking into consideration that much longer time (24 h) was required for most substrates to fully transfer into the final products, and the identical enantiopurity of 6 and that of 2a obtained under the standard conditions, we proposed that the stereochemistry of the whole reaction is established irreversibly in the aminative dearomatization step, whereas the following Michael addition is the rate-limiting step. Fig. 4 Isolation of the Intermediate. Reaction conditions: 1a (0.1 mmol), DEAD (0.15 mmol) and ( S )- C2 (10 mol%) in DCE (2 mL) at 50 °C for 30 min Full size image To explore the origin of the exceedingly high enantioselectivity, DFT calculations were then performed for the aminative dearomatization step (Fig. 5 ). The relative Gibbs free energy of TS-major , the transition state leading to the major product, was 2.0 kcal/mol lower than that of TS-minor , which was in qualitative agreement with the experimental results. The two prochiral faces at the C4 position of α -naphthol were well discriminated by the chiral phosphoric acid. In TS-major , the Si -face of the C4 position was attacked, which allowed the intact benzene ring of α -naphthol in distal to the chiral pocket. Whereas in TS-minor , strong steric congestion was developed due to the Re -face attack and the concomitant approximation of the intact benzene ring to one TRIP group of C2 . 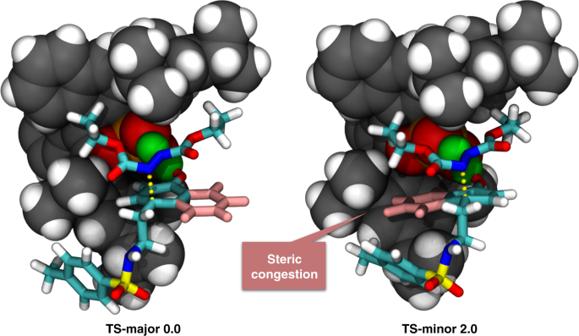Fig. 5 Transition states. Optimized structures and relative Gibbs free energies (in kcal/mol) of the transition states of the aminative dearomatization step (ωB97XD/def2-TZVPP//B97D/6-31G**). The catalysts are presented with the van der Waals model. The substrates are presented with the stick model. The forming C–C bonds are shown in yellow dash lines. The transferring protons are shown in green spheres. The intact benzene rings ofα-naphthols are shown in pink 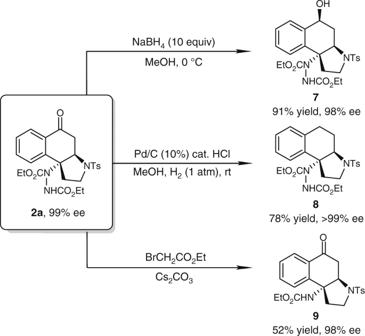Fig. 6 Transformations of2a. Reaction conditions for synthesis of7:2a(0.2 mmol), NaBH4(2.0 mmol) in MeOH (4 mL) at 0 °C. Reaction conditions for synthesis of8:2a(0.2 mmol), Pd/C (10%, 50 mg), HCl (conc. 20 μL) in MeOH (4 mL) under H2(1 atm) at room temperature. Reaction conditions for synthesis of9:2a(0.2 mmol), Cs2CO3(0.26 mmol), BrCH2CO2Et (0.22 mmol) in CH3CN (4 mL) at 50 °C These computational results corresponded well with the fact that substituents were tolerated at the C6 to C8 positions of α -naphthol ( 2k–2u ), but not at the C2 position ( 2v ). In addition, a fused saturated skeleton that is sterically roughly comparable with a benzene ring should be beneficial for the high enantioselectivity ( 4a ), but sterically less demanding 2,3-Me 2 groups were not that effective ( 4b ). Fig. 5 Transition states. Optimized structures and relative Gibbs free energies (in kcal/mol) of the transition states of the aminative dearomatization step (ωB97XD/def2-TZVPP//B97D/6-31G**). The catalysts are presented with the van der Waals model. The substrates are presented with the stick model. The forming C–C bonds are shown in yellow dash lines. The transferring protons are shown in green spheres. The intact benzene rings of α -naphthols are shown in pink Full size image Product transformations To highlight the practicality and synthetic utility of this method, a gram-scale reaction of 1a with DEAD was performed under the standard reaction conditions. 2a was obtained in 87% yield (1.35 g) with 99% ee. In addition, several functional group transformations of 2a were demonstrated (Fig. 6 ). Tertiary alcohol 7 was delivered in 91% yield when treated with NaBH 4 . The ketone group could also be hydrogenated to methylene group under the catalysis of palladium on charcoal, leading to 8 in 78% yield. In addition, the N–N bond could be cleaved by treating 2a with ethyl bromoacetate and cesium carbonate. The corresponding product 9 was afforded in 52% yield. Notably, no erosion of enantiomeric purity was observed in all these transformations. Fig. 6 Transformations of 2a . Reaction conditions for synthesis of 7 : 2a (0.2 mmol), NaBH 4 (2.0 mmol) in MeOH (4 mL) at 0 °C. Reaction conditions for synthesis of 8 : 2a (0.2 mmol), Pd/C (10%, 50 mg), HCl (conc. 20 μL) in MeOH (4 mL) under H 2 (1 atm) at room temperature. Reaction conditions for synthesis of 9 : 2a (0.2 mmol), Cs 2 CO 3 (0.26 mmol), BrCH 2 CO 2 Et (0.22 mmol) in CH 3 CN (4 mL) at 50 °C Full size image In conclusion, we have achieved a chiral phosphoric acid-catalyzed dearomatization reaction of α -naphthols bearing a tethered nucleophile at the C4 position of the naphthol ring. Preliminary mechanistic investigations confirmed that the reaction proceeded via two steps, a stereochemistry-determining aminative dearomatization followed by a rate-limiting Michael addition. The reaction occurred under mild conditions, affording a wide array of polycyclic ketones in good yields with excellent enantioselectivity. Besides, the reaction features high catalytic efficiency and diverse transformations of the products. A working model accounting for the origin of the stereochemical induction was proposed based on DFT calculations. Representative procedure To a flask containing a mixture of 1a (0.1 mmol) and ( S )- C2 (7.5 mg, 0.01 mmol) under argon was added a solution of the corresponding azodicarboxylate (0.15 mmol) in anhydrous 1,2-dichloroethane (2 mL). The reaction was stirred at 50 °C until TLC showed complete consumption of the starting material. The reaction mixture was cooled to room temperature, quenched with NaHCO 3 (aq., 10 mL) and extracted with CH 2 Cl 2 (3 × 15 mL). The combined organic layer was washed with brine, separated, dried over Na 2 SO 4 and filtrated. After the solvent was removed under reduced pressure, the residue was purified by silica gel column chromatography (ethyl acetate/petroleum ether = 1/6 to 1/2) to afford 2a .